Larger mitochondrial DNA than Y-chromosome differences between matrilocal and patrilocal groups from Sumatra Genetic differences between human populations are typically larger for the Y-chromosome than for mitochondrial DNA (mtDNA), which has been attributed to the ubiquity of patrilocality across human cultures. However, this claim has been disputed, and previous analyses of matrilocal groups give conflicting results. Here we analyse mtDNA variation (complete mtDNA genome sequences via next-generation sequencing) and non-recombining regions of the Y-chromosome variation (Y-single-nucleotide-polymorphisms and Y-short-tandem-repeats (STR)) in a matrilocal group (the Semende) and a patrilocal group (the Besemah) from Sumatra. We find in the Semende significantly lower mtDNA diversity than in the Besemah as expected for matrilocal groups, but unexpectedly we find no difference in Y-chromosome diversity between the groups. We highlight the importance of using complete mtDNA sequences for such analyses, as using only partial sequences (as done in previous studies) can give misleading results. The extent to which cultural practices influence human genetic diversity has been a longstanding question in anthropological genetics. Genetic differences between human populations are usually larger for non-recombining regions of the Y-chromosome (NRY) than for mitochondrial DNA (mtDNA) [1] , [2] , [3] , and this pattern has been attributed to higher female than male migration due to patrilocality [1] , [4] , which is typical for about 70% of human societies [5] . Higher female than male migration results in a larger effective population size for females than males, which in turn predicts increased mtDNA and decreased Y-chromosome diversity within groups, and larger differences between groups for the Y-chromosome than for mtDNA. An obvious test of this hypothesis is that the genetic differences among matrilocal groups should then be larger for mtDNA than for the NRY and that the mtDNA diversity is lower in matrilocal groups than patrilocal. Indeed, this prediction was fulfilled in the first comparison of patterns of mtDNA and NRY variation in matrilocal and patrilocal groups, among the hill tribes of Thailand [4] , [6] . However, a subsequent study of matrilocal and patrilocal groups in India failed to find the predicted patterns of mtDNA versus NRY diversity [7] , whereas another study has called into question the original observation of larger differences among human groups in general for the NRY versus mtDNA [8] . Clearly, studies of additional matrilocal groups are needed to ascertain if there is a general effect of residence pattern on human mtDNA and NRY diversity. We report here an analysis of complete mtDNA genome sequences (determined by next-generation sequencing) and NRY haplogroups and Y-STR haplotypes in a matrilocal group (the Semende) and a patrilocal group (the Besemah) from Sumatra, Indonesia. With respect to mtDNA, we find a lower haplotype diversity (HD) in the Semende, and a significantly large genetic distance between the Semende and the Besemah, as expected if matrilocality is influencing patterns of mtDNA diversity. Unexpectedly, and in contrast to virtually every other study of human mtDNA versus NRY diversity on the local scale, there are no significant differences between these two groups for the NRY. Moreover, our results highlight the importance of obtaining complete mtDNA genome sequences, as there are no significant differences in HD between the Besemah and Semende when only partial sequences are analysed, as was done in previous studies [7] , [8] . mtDNA sequences We obtained 36 complete mtDNA sequences from the Semende (a matrilocal group) and 36 from the Besemah (a patrilocal group) from Sumatra, Indonesia, using high throughput, parallel tagged sequencing [9] , [10] on the Roche GS/FLX (Roche) and Illumina GAII platforms (Illumina). Sequences were assigned to the closest haplogroup for which all defining mutations were present. For both groups, 24 mtDNA haplogroups were observed ( Fig. 1 ), of which 7 belong to macrohaplogroup M ( Supplementary Fig. S1 ) and 17 to macrohaplogroup N ( Supplementary Fig. S1 ). The majority of the sequences from the Semende (44%) belong to the basal haplogroups M1′51 and a new haplogroup, M*. 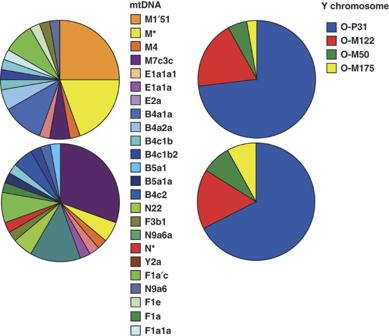Figure 1: mtDNA and NRY haplogroup frequencies for the Semende and the Besemah. Haplogroup composition and frequencies based on complete mtDNA sequences and Y-SNPs. For the Besemah, haplogroup M7c3c was at the highest frequency (31%), followed by haplogroup E1a1a at a frequency of 14% ( Table 1 ). Figure 1: mtDNA and NRY haplogroup frequencies for the Semende and the Besemah. Haplogroup composition and frequencies based on complete mtDNA sequences and Y-SNPs. Full size image Table 1 Haplogroup frequencies for mtDNA. 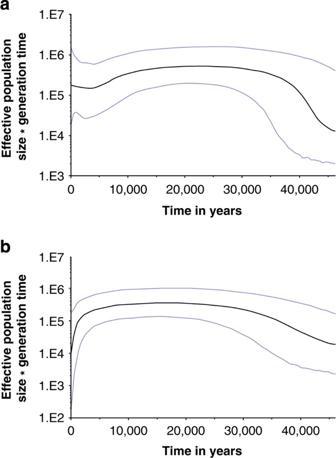Figure 2: Bayesian Skyline Plots of effective population size through time. BSP based on the mtDNA coding region, estimated with 30 million MCMC iterations and sampled every 3,000 steps. Theyaxis for each plot is the product of the effective population size and the generation time and thexaxis shows time. A mutation rate of 1.69×10−8per site per year49was used. (a) BSP for Besemah, using all 36 sequences. (b) BSP for Semende, using all 36 sequences. Full size table The mtDNA HD for the complete mtDNA genomes ( Table 2 ) is lower in the Semende than in the Besemah, and the difference is highly significant by a permutation test ( P <0.001) ( Supplementary Fig. S2 ). Conversely, the mean number of pairwise differences ( Table 2 ) was significantly higher ( P <0.03, Supplementary Fig. S2 ) in the Semende ( k =36.18) than in the Besemah ( k =32.34). Furthermore, the F ST value for the mtDNA is 0.076 and is significantly different from 0 ( P =0). As a previous study that failed to find a difference in patterns of mtDNA diversity between matrilocal and patrilocal groups in India only sequenced the HV1 region [7] , we also analysed only the HV1 sequences from the Semende and Besemah. In contrast to the results based on complete mtDNA genome sequences, the difference in mtDNA HD is not significant between the Semende and Besemah ( Supplementary Fig. S2 ), but the mean number of pairwise difference is significantly higher in the Semende than Besemah ( P <0.01). Likewise, the F ST value is 0.088 and is significantly different from 0 ( P =0). Table 2 Summary statistics for the mtDNA and Y-chromosome. Full size table To further investigate the maternal history of the Semende and the Besemah, we carried out a Bayesian analysis of changes in population size through time [11] . The Bayesian Skyline Plots (BSPs), based on the complete mtDNA genome sequences, differ between the two groups: the Besemah exhibit a steep increase in population size beginning around 40,000 years ago and a slight decrease around 10,000 years ago ( Fig. 2a ), whereas the Semende show a more gradual increase beginning around 40,000 years ago, and a sharp decrease beginning around 5,000 years ago ( Fig. 2b ). The BSPs also indicate that the current estimated effective population size of the Semende is about ten times lower than that of the Besemah. Figure 2: Bayesian Skyline Plots of effective population size through time. BSP based on the mtDNA coding region, estimated with 30 million MCMC iterations and sampled every 3,000 steps. The y axis for each plot is the product of the effective population size and the generation time and the x axis shows time. A mutation rate of 1.69×10 −8 per site per year [49] was used. ( a ) BSP for Besemah, using all 36 sequences. ( b ) BSP for Semende, using all 36 sequences. Full size image NRY variation Y-single-nucleotide polymorphisms (SNPs) and Y-STRs were typed for all individuals, however results could not be obtained for all STR loci for one Besemah, who therefore was excluded from the Y-STR analysis. The Y-SNP haplogroup for each individual and the Y-STR haplotypes are provided in Supplementary Table S1 . Only four NRY haplogroups were observed for both groups, and all individuals belonged to haplogroup O or sublineages thereof ( Fig. 1 ). Both groups had high frequencies of O2 (O-P31) (>70%) and O3 (O-M122) (16–19%), whereas haplogroups O1a2 (O-M50) and O* were found at low frequencies in both groups ( Table 3 ). In contrast to the mtDNA results, the distribution of Y-SNP haplogroups is very similar in the two groups ( Fig. 1 ) and does not differ significantly ( P >0.05). Moreover, the F ST value for Y-STRs between the Semende and Besemah is only 0.013, and is not significantly different from 0 ( P >0.05). Network analysis showed that Y-STR haplotypes are also shared to a large extent between the two groups ( Supplementary Fig. S3 ). Neither HD values nor mean number of pairwise differences ( k ), based on Y-STRs, differ significantly between the Semende (HD=0.95, k =5.65) and the Besemah (HD=0.93, k =5.52), based on permutation tests ( Supplementary Fig. S2 ). Table 3 Y-chromosome haplogroup frequencies. Full size table If residence pattern influences genetic diversity, then mtDNA HD is expected to be lower in matrilocal than patrilocal groups. This is indeed the case ( Table 2 ): mtDNA diversity is significantly lower (as judged by a permutation test; Supplementary Fig. S2 ) in the matrilocal Semende than in the patrilocal Besemah. Interestingly, the HD of the HV1 in the Besemah is lower, but not significantly so. No other studies looking at genetic diversity differences between patrilocal and matrilocal groups have used complete mtDNA sequences before; most studies have used only part of the mtDNA genome, usually HV1. These results indicate that it may be insufficient to use only the HV1 to make inferences concerning genetic variation and differences. In particular, perhaps the failure of identifing such differences in previous studies is due to the lack of power using only the HV1 (ref. 7 ) or only a single gene such as MT-CO3 (ref. 8 ). The higher mean number of pairwise differences in the matrilocal group probably reflects the very different haplogroup composition of this group ( Fig. 1 and Table 1 ): around 20% of mtDNA lineages in the Semende belong to a new haplogroup M* restricted to this population and another 25% belong to a new subgroup of M1′51. This new subgroup of M1′51 shares 12 mutations with M51 ( Supplementary Fig. S1 ), a recently described haplogroup found in one Cambodian individual [12] . M1′51 is basal to subgroups found in North and West Africa and South Europe and is believed to have arisen in southwestern Asia and to have been brought back to Africa and South Europe via a back-migration [13] . Except for the one Cambodian individual, no other subgroups of M1′51 have been found before in Asia to date. The rest of the mtDNA lineages in the Semende belong to 13 different haplogroups ( Fig. 1 ). Altogether, 53% of the sequences belong to haplogroups frequently found in West and Southeast Asia, for example, subclades of haplogroups B4, B5, R9 and N9 (refs 14 , 15 , 16 ). In the Besemah, the mtDNA lineages fall into 17 different haplogroups ( Fig. 1 and Table 2 ); 95% of their mtDNA haplogroups have been previously described in West and Southeast Asia (with some variation at the tips of the branches), including subhaplogroups of N9, M7, F1, E1, E2, B4 and B5 (refs 14 , 15 , 16 ). Haplogroup M7c3c has the highest frequency (31%), followed by E1a1a (14%) which are both widespread and found at high frequencies in Southeast Asia [14] , [15] , [17] . The Besemah also have one unique M* lineage; one sample with the same haplotype as two M* Semende sequences; one sequence that branches off haplogroup M4; and one N* lineage that shares some mutations with N21 ( Supplementary Fig. S1 ). The M4 lineage shares some mutations with the M4 lineage from the Semende, but each have several unique mutations. Subgroups of M4 have been previously reported in tribal populations in India [18] , [19] , Nepal [20] and in the Philippines [21] . There is thus a striking dichotomy in the mtDNA lineages between the matrilocal Semende and the patrilocal Besemah. The Semende have high frequencies of M* and M1′51 lineages not found elsewhere in the world to date, which suggests that these lineages have been maintained in the matrilocal population, perhaps through matrilocal practices, for a long time. By contrast, the majority of the mtDNA lineages in the Besemah are found at high frequency in Southeast Asia and indicate that there has been substantial mtDNA gene flow between this group and surrounding groups, as expected in patrilocal societies. To further investigate the observed differences in mtDNA diversity, we generated BSPs based on the coding region of the mtDNA genomes ( Fig. 2 ). The BSPs indicate that the matrilocal group has a lower effective population size than the patrilocal group, as expected from their lower genetic diversity. Furthermore, the BSPs indicate different histories for these groups: the Besemah show signatures of population expansion, followed by a slight population reduction, whereas the population size has been relatively more constant for the Semende, with a recent steep population reduction. Unexpectedly, patterns of NRY variation are very similar, and do not differ significantly, between the two groups. Haplogroup O2 has the highest frequency in both groups (>70%), and this haplogroup is found at high frequency in Southeast Asia [22] , [23] , and it's subhaplogroup O2a (O-M95) in Indonesia [24] . Haplogroups O3 (O-M122) and O1a (O-M119), which are found at low frequency in both groups, have been associated with the Austronesian expansion and are found at high frequency throughout Southeast Asia [22] , [23] , [25] . These results are surprising, as other studies have shown that, in general, there is more structure within human populations for Y-chromosome diversity than for mtDNA, which is likely to reflect the high global prevalence of patrilocality [1] , [5] . Furthermore, patrilocal practises seem to be more tightly regulated than matrilocal practices [4] , resulting in a higher female than male migration rate [2] , [26] , [27] , [28] . Perhaps matrilocality has been more tightly regulated in the Semende, and patrilocality less tightly regulated in the Besemah, than has been observed previously. The similarity in NRY diversity for these groups could also be explained by a recent conversion to patrilocality of the Besemah. The current matrilocal and patrilocal residence patterns of the Besemah and Semende are documented since the middle of the 19th century [29] , [30] , [31] , but it is unknown when they were first established. It has been hypothesized that matrilocality is ancestral in Austronesian societies and that descendant groups of Austronesian people in the Pacific adopted a patrilocal residence pattern over time, as a switch from matrilocality to patrilocality is more common than the reverse change [32] . A relatively recent change to patrilocality of the Besemah would explain the low frequency of unique mtDNA lineages as those would have been replaced by new, incoming lineages. The lack of unique NRY types can likewise be explained by a former practise of matrilocality for which inmarrying men would have continuously introduced new Y-chromosomes. The original residence pattern is expected to be reflected in patterns of genetic variation at least 5–6 generations after any switch [28] , but to have disappeared after about 20 generations [33] . Therefore, if the Besemah were previously a matrilocal group, the switch to patrilocality must have happened at least 150 years ago (assuming a generation time of 25 years for females), but not so long ago that there has been time for patterns of NRY variation to reflect the switch to patrilocality. However, differences in resolution for mtDNA versus the Y-chromosome may also have a role, as we have more detailed information for mtDNA (the complete sequence, compared with a few Y-SNPs and Y-STRs). In conclusion, it is highly likely that the unique M* and M′51 mtDNA lineages present in the Semende reflect the initial settlement of the region, and that matrilocality has preserved these lineages. By contrast, patterns of Y-chromosome diversity do not differ between the Besemah and the Semende, suggesting that local groups were more heavily influenced by male gene flow from expanding populations. Notably, the significant differences in mtDNA HD between the Besemah and Semende were only revealed by the complete mtDNA genome sequences, and not by HV1 sequences alone. Thus, previous studies that analysed only a portion of the mtDNA genome and failed to find a difference relating to matrilocality versus patrilocality may have lacked sufficient resolution. Overall, our results confirm the idea that cultural practices can influence genetic variation [34] , but also demonstrate that the expected influence of matrilocality and patrilocality on genetic diversity may not always hold; in particular, in the present case, matrilocality seems more tightly regulated than patrilocality, in contrast to previous results [4] . DNA samples Saliva samples were collected with informed consent by Hengky Firmansyah from nine locations in Sumatra, Indonesia ( Supplementary Table S2 ), consisting of 38 samples from the Besemah (a patrilocal group) and 37 from the Semende (a matrilocal group). DNA was extracted as described previously [35] . These agricultural groups live in very close proximity to each other and are linguistically similar, speaking closely related dialects that are partially mutually intelligible (David Gil, field observation). All samples were collected in villages close to Pagaralam except one that was collected in Padang. The use of these samples in this research was approved by the Ethics Commission of the University of Leipzig Medical Faculty. MtDNA genome sequencing Complete mtDNA genome sequences were obtained for 36 samples from each group, 27 with the Roche GS/FLX platform (Roche) and 45 with the Illumina GAII platform (Illumina; Supplementary Table S2 ); coverage for three samples was too low for subsequent analysis and hence these were excluded. All libraries sequenced with the GS/FLX and 12 samples that were sequenced with the GAII were prepared from long-range PCR products. Two overlapping long-range PCR products were amplified for the sequencing of the complete mtDNA genome using primers described previously [21] . The libraries for the remaining 33 samples were prepared using a targeting method designed for the Genome Analyzer platform in which each individual is given its own barcode during the library preparation [10] . The samples were then enriched with a capture method in which mtDNA PCR products were used to capture library mtDNA templates [36] . These samples were sequenced on the GAII analyzer with single reads and 76 cycles (see Supplementary Table S2 for more details). Assembly of the sequences was carried out with a mapping iterative assembler as described previously [37] , using the revised Cambridge Reference Sequence (rCRS) as a reference to which all reads were mapped. A multiple alignment was performed with mafft v6.708b [38] . For the consensus sequences obtained from the mapping iterative assembler, all bases were covered at least two times (bases with <2× coverage were replaced with N's, as missing data; see Supplementary Table S2 for the number of N's in each sequence). A maximum of 1% missing data (N's) was accepted; the number of N's per sequence ranged from 0 to 26 ( Supplementary Table S2 ). Overall, the average coverage was 54-fold, ranging from 9 to 144 with an average minimum coverage of 15.5 ( Supplementary Fig. S4 and Supplementary Table S2 ). Sequences were manually checked and edited because of homopolymer problems occuring with the GS/FLX technology. This problem stems from the inaccuracy in the light signal intensity resulting from runs of three or more identical bases, making it impossible to detect the exact number of bases in such homopolymer regions [39] . Therefore, sequences were manually checked and edited and insertions or deletions were removed in a homopolymer run in a genic region, but not in non-coding regions. These edited positions never occurred at a polymorphic, biallelic site, and all indels were not used in subsequent analyses. These manually edited sequences have been submitted to GenBank (accession numbers: HM596644 to HM596715 ). NRY genotyping A total of 12 Y-SNPs (C-RPS4Y, C-M38, C-M208, M-M4, M-P34, M-M104, K-M9, NO-M214, O-M119, O-M122, P-M74, R-M173) were typed using a single-base extension assay with amplicons detected by matrix-assisted laser desorption ionization time-of-flight mass spectrometry using methods described elsewhere [40] . For a higher resolution of specific Y-chromosome haplogroups, further Y-SNPs were detected by hierarchic multiplexes [41] and genotyping performed with the ABI Prism SnaPshot multiplex kit (Applied Biosystems), with amplicons detected using capillary electrophoresis on an ABI Prism 3100 Genetic Analyzer according to the manufacturer's instructions. Hierarchical SNP typing was done in two SnaPshot multiplexes; in the first one six SNPs were typed (O-M175, M-M5, O-M122, O-P31, N-LLy22g and O-M134), whereas in the second one three SNPs were typed (O-119, O-M101 and O-M50). In addition, 12 Y-STR loci (DYS391, DYS389I, DYS439, DYS389II, DYS438, DYS437, DYS29, DYS392, DYS393, DYS390, DYS385a, DYS385b) were typed using the Promega PowerPlex Y system (Promega Corporation) with amplicons detected on an ABI Prism 3100 Genetic Analyzer (Applied Biosystems), all following the manufacturer's instructions. The phylogenetic relationship of the complete set of SNPs typed in the study is shown in Supplementary Figure S5 , following the nomenclature of they Y-chromosome phylogenetic tree [42] . Data analysis The mtDNA genome sequences were assigned to haplogroups according to Phylotree.org Build 7 [43] using a custom Perl script. Positions 309.1C(C), 16182C, 16183C, 16193.1C(C) and 16519 were not used for haplogroup assignment as these are subject to highly recurrent mutations. Y-chromosome haplogroup affiliations were based on the YCC tree [42] . Basic descriptive diversity statistics were calculated with dnaSP v5 for the complete mtDNA sequences. The Arlequin software package [44] , version 3.5 was used to calculate summary statistics for the NRY data. To test if the diversity values (HD and the mean number of pairwise differences) differed significantly between groups, a custom R script ( Supplementary Software ) was used to perform a permutation test in which the complete dataset was split randomly into two populations 1,000 times and the relevant diversity statistic was calculated each time, and then the difference between the two randomly generated groups was calculated and compared with the difference between the values obtained from the observed data. The same approach was used to test whether the mean number of pairwise differences ( k ) for the mtDNA data was significantly different between groups, using the function dist.dna from the R package APE [45] . As APE only deals with sequence data, a custom R script was used to do the same test based on the mean number of pairwise differences for the Y-STR data. Before performing the permutation tests, all sites with indels and missing data (N's) were deleted, except for two indel sites, which were recoded as base substitutions as follows: the 9 bp deletion in the intergenic region between the MT-CO2 and lysine tRNA genes was coded as a transitional difference (9-bp deletion=T, absence of deletion=C); and the CA microsatellite beginning at position 520 (five repeats=A, four repeats=T, three repeats (only in one case)=G). In total, 132 sites were deleted, or 0.8%. As this dataset was used for the permutation test, all summary statistics were calculated using this dataset in dnaSP. The mtDNA coding region (positions 577–16,023) was used to generate BSPs using Markov chain Monte Carlo (MCMC) sampling in the program BEAST (version 5.1) [46] , [47] , using the same parameters as described previously [21] . Each run was analysed using the program Tracer for independence of parameter estimation and stability of MCMC chains [47] . Network analyses [48] were carried out using version 4.516 of Network and version 1.1.0.7 of Network Publisher. Networks for Y-STR haplotypes used a weighting scheme based on Y-STR locus-specific mutation rates obtained from NIST ( http://www.cstl.nist.gov/biotech/strbase/ ). Data deposition : The complete consensus mtDNA sequences were submitted to GenBank Nucleotide Core database under accession numbers HM596644 to HM596715 . How to cite this article: Gunnarsdóttir, E.D. et al . Larger mitochondrial DNA than Y-chromosome differences between matrilocal and patrilocal groups from Sumatra. Nat. Commun. 2:228 doi: 10.1038/ncomms1235 (2011).